Genome-wide association and high-resolution phenotyping linkOryza sativapanicle traits to numerous trait-specific QTL clusters Rice panicle architecture is a key target of selection when breeding for yield and grain quality. However, panicle phenotypes are difficult to measure and susceptible to confounding during genetic mapping due to correlation with flowering and subpopulation structure. Here we quantify 49 panicle phenotypes in 242 tropical rice accessions with the imaging platform PANorama. Using flowering as a covariate, we conduct a genome-wide association study (GWAS), detect numerous subpopulation-specific associations, and dissect multi-trait peaks using panicle phenotype covariates. Ten candidate genes in pathways known to regulate plant architecture fall under GWAS peaks, half of which overlap with quantitative trait loci identified in an experimental population. This is the first study to assess inflorescence phenotypes of field-grown material using a high-resolution phenotyping platform. Herein, we establish a panicle morphocline for domesticated rice, propose a genetic model underlying complex panicle traits, and demonstrate subtle links between panicle size and yield performance. As the bearers of grain, grass inflorescences have been the target of selection for thousands of years [1] . In Asian rice ( Oryza sativa ), a staple crop for billions of people, optimizing rice panicle size and structure represents a challenge for breeders attempting to improve yield potential and maximize grain quality [1] , [2] . Panicle size and branching patterns in rice have increased in complexity throughout domestication and modern breeding; however, when compared to its wild ancestors, it is clear that changes in O. sativa panicle architecture have been relatively subtle. Seeds are born on long primary branches that sometimes iterate into secondary and tertiary branches [2] , [3] , and although phenotypes are often variety specific, they are also variable under different environmental conditions [3] , [4] , [5] . Meristematic transitions during panicle development are spatiotemporally regulated, affecting the number and position of rice grains, as well as grain filling rate and seed quality [6] , [7] . Thus, unlike in maize ( Zea mays ), where inflorescences have been selected for extreme divergence into a branchless female cob and a highly branched male tassel [8] , panicles from many modern rice varieties still resemble those from their closest wild relatives, Oryza rufipogon and Oryza nivara [9] . Many genes have been cloned relating to rice inflorescence development [6] , [10] , several of which are agronomically important. The OsLIGULESS1 ( OsLG1 ) locus was recently identified as a domestication gene and controls the shift from open to closed panicles [11] . A natural allele of DENSE AND ERECT PANICLE 1 ( DEP1 ) within high-yielding Chinese rice varieties boosts yield potential by pleiotropically reducing panicle internode length (NL), while increasing both primary and secondary branch number [12] . In addition, a major effect allele for Grain Number 1a ( GN1a ) significantly increases secondary panicle branching, grain count and yield [13] , and is already being incorporated into breeding pipelines. However, although many studies have examined the role of candidate genes in the reference sequenced variety (Nipponbare) or a few close relatives, panicle architecture has not been characterized in detail across diverse varieties grown in field conditions. The inbreeding nature of rice and multiple origins of domestication have led to the formation of deep subpopulation structure, which has partitioned genetic and phenotypic variation in the species. O. sativa comprises two major varietal groups (sometimes referred to as subspecies), Indica and Japonica , which can be further divided into five subpopulations ( indica , aus , tropical japonica , temperate japonica and aromatic/Group V ) [14] , [15] , [16] . Several genome-wide association studies (GWASs) have confirmed that variation exists both within and between rice subpopulations for important agronomic traits [16] , [17] , [18] , [19] , [20] , including panicle count and panicle length (PL) [16] , [19] . However, low-resolution panicle phenotyping has probably limited the ability to accurately assess genetic architecture of panicle traits [21] . In this study, we performed GWAS using phenotypes collected with a high-resolution panicle phenotyping platform, PANorama [21] , and a genotypic data set of 700,000 single-nucleotide polymorphisms (SNPs) assayed using a high-density rice array (HDRA) [20] . Unlike previous studies, which focused on collecting a few trait measurements in a large population of accessions [16] , [17] , we collected a large number of panicle and agronomic phenotypes on a targeted population of 242 diverse rice accessions grown under field conditions in the Philippines. Using phenotypic covariates within the GWAS model to examine relationships among traits, we identify a large number of GWAS peaks associated with panicle size, suggest pleiotropic relationships between panicle traits and link several candidate genes to rice panicle development. We validate these associations using quantitative trait loci (QTL) mapping in a recombinant inbred line (RIL) population and demonstrate that panicle traits share subtle relationships with other important agronomic traits, phenotypically and genotypically. 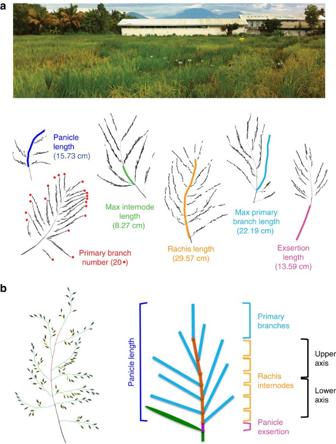Figure 1: Panicle phenotyping inO. sativa. (a) A diverse collection of landraces were assessed for panicle and agronomic traits under field conditions. Photographs from different accessions with extreme panicle phenotypes, depicted in relative scale, highlight the range of phenotypic diversity within the panel. (b) The PANorama phenotyping platform generates skeletons (left) from panicle images using exact morphological erosions of shapes. The schematic depicts the major classes of phenotypes extracted from panicle skeletons (right). Diversity panel selection and population structure The phenotyping panel in this study contained 242 inbred rice varieties, most of which are tropically or subtropically adapted accessions, and represented germplasm from 60 countries ( Supplementary Table 1 ). Using the Bayesian clustering software fastStructure [22] , we calculated varying levels of K means ( Supplementary Fig. 1a ). The Indica and Japonica varietal groups appear clearly at K =2, and at K =3 Indica further divides into the indica and aus subpopulations. Using principle component (PC) analysis, we confirmed that the top three PCs account for the aus , indica and tropical japonica subpopulations and explain ∼ 30% of the genetic variation within our panel ( Supplementary Fig. 1b ). The optimal number of subpopulations was predicted to be K =8, based on model complexity and model component analysis as computed by fastStructure [22] . Although K =7 or K =8 clearly defined variation within and between indica , aus , tropical japonica , temperate japonica and admixed accessions, we used the first three PCs as covariates within the GWAS model to control for subpopulation structure (see Methods and Supplementary Fig. 1 ). These results are consistent with previous studies quantifying the population structure of O. sativa and confirm that our panel captures abundant genetic variation in tropical rice germplasm [15] , [17] , [19] , [23] . Novel phenotyping reveals rice panicle trait relationships Using the image skeletonization phenotyping platform PANorama [21] , we measured 49 phenotypes from over 3,400 images of rice panicles collected in the field ( Fig. 1a ). Width, length and count phenotypes were extracted from images by subdividing panicles into nested measurements of three major panicle traits: primary branches, rachis internodes and the peduncle above the flag leaf ligule, also referred to in rice as panicle exsertion [24] , which is a measurement of the uppermost internode of the panicle-bearing culm ( Fig. 1b ). Several novel, nested measurements were incorporated into PANorama and are available in an updated version of the open-source software (Methods). We also collected 11 vegetative and reproductive stage phenotypes, including a measurement of flowering time (heading date (HD)). 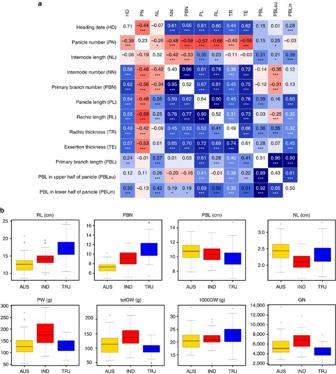Figure 2: Phenotypic analysis reveals trait relationships and subpopulation characteristics. (a) A heatmap depicting Pearson’s correlation coefficients between phenotype means (lower triangle) and genetic best linear unbiased predictors (GBLUPs) (upper triangle) for a subset of traits across all varieties within the study. AD heritabilities are located within the diagonal. Trait acronyms are in parentheses. Asterisks indicate significant correlations using a two-tailedt-test (**P<0.001 and ***P<0.0001) andn=242 varieties. All pairwise comparisons between traits are inSupplementary Figs 3 and 4. (b) Phenotypic distributions of panicle and agronomic traits, divided by theaus(AUS),indica(IND) andtropical japonica(TRJ) subpopulations: RL, PBN, PBL, NL, panicle weight (PW), total grain weight (totGW), 1,000GW and grain number (GN). Within boxplots, the bold line represents the median, box edges represent upper and lower quantiles, and whiskers are 1.5 times the quantile of the data. Outliers are shown as open dots. The number of varieties within each subpopulation was as follows: panicle traits (63aus, 84indica, 79tropical japonica) and yield traits (34aus, 51indicaand 45tropical japonica). Detailed descriptions of each phenotype are presented in Supplementary Table 2 . Figure 1: Panicle phenotyping in O. sativa . ( a ) A diverse collection of landraces were assessed for panicle and agronomic traits under field conditions. Photographs from different accessions with extreme panicle phenotypes, depicted in relative scale, highlight the range of phenotypic diversity within the panel. ( b ) The PANorama phenotyping platform generates skeletons (left) from panicle images using exact morphological erosions of shapes. The schematic depicts the major classes of phenotypes extracted from panicle skeletons (right). Full size image As the diversity panel comprises inbred accessions and does not contain heterozygous alleles, it was not possible to calculate true heritabilities for each phenotype; instead, we estimated narrow sense ( h 2 ) heritability by calculating additive+dominance (AD) heritability [25] and broad sense (H) heritability by calculating repeatability between raw phenotypes (Methods). For some traits, AD and H heritabilities were nearly equivalent, demonstrating the power of image analysis in reducing measurement error ( Supplementary Fig. 2 ). We also calculated genetic correlation among phenotypes and compared it with phenotype × phenotype correlations (see Methods and Supplementary Figs 3 and 4 ). In general, phenotypic and genotypic correlations among panicle traits mirrored one another and were highly significant ( Fig. 2 ); the median Pearson’s correlation coefficient between pairwise phenotypes was r= 0.4. Increases in width traits such as rachis thickness and exsertion thickness were positively correlated with increased primary branch length (PBL) and primary branch number (PBN). Internode number (NN) and PBN, which estimate meristematic divisions, were positively correlated ( Fig. 2a ). Groups of sub-traits were tightly correlated, such as the nested phenotypes PBL in the lower and upper halves of the panicle (PBLin versus PBLsu) ( Figs 1b and 2 and Supplementary Figs 3 and 4 ). In short, larger panicles always showed thicker axes, longer branches and higher counts of branches and internodes. Figure 2: Phenotypic analysis reveals trait relationships and subpopulation characteristics. ( a ) A heatmap depicting Pearson’s correlation coefficients between phenotype means (lower triangle) and genetic best linear unbiased predictors (GBLUPs) (upper triangle) for a subset of traits across all varieties within the study. AD heritabilities are located within the diagonal. Trait acronyms are in parentheses. Asterisks indicate significant correlations using a two-tailed t -test (** P <0.001 and *** P <0.0001) and n =242 varieties. All pairwise comparisons between traits are in Supplementary Figs 3 and 4 . ( b ) Phenotypic distributions of panicle and agronomic traits, divided by the aus (AUS), indica (IND) and tropical japonica (TRJ) subpopulations: RL, PBN, PBL, NL, panicle weight (PW), total grain weight (totGW), 1,000GW and grain number (GN). Within boxplots, the bold line represents the median, box edges represent upper and lower quantiles, and whiskers are 1.5 times the quantile of the data. Outliers are shown as open dots. The number of varieties within each subpopulation was as follows: panicle traits (63 aus , 84 indica , 79 tropical japonica ) and yield traits (34 aus , 51 indica and 45 tropical japonica ). Full size image High-resolution phenotyping captured several novel relationships among traits. Inverse correlations between length and count traits have been well documented in rice, especially between panicle number and panicle size ( Fig. 2 and Supplementary Figs 3 and 4 ), highlighting physiological and physical tradeoffs during development [7] , [26] . Although NL had a strong negative correlation with NN ( r =−0.42), NL was weakly correlated with rachis length (RL) ( Fig. 2 and Supplementary Figs 3 and 4 ), suggesting that increased NN is more important than NL in driving increases in overall panicle size. Surprisingly, PBL and PBN phenotypes were not significantly correlated or showed minimal positive correlation. PBL in the upper (PBLsu) and lower (PBLin) halves of the panicle ( Fig. 1b ) also had different phenotypic and genetic relationships with PBN and NN, which is consistent with previous evidence for differential protein expression in spikelets on the upper and lower halves of the panicle [27] ( Fig. 2 and Supplementary Figs 3 and 4 ). Panicle phenotypes also showed distinct distributions within subpopulations ( Fig. 2b ). The tropical japonica subpopulation had the highest average RL (17 cm) and PBN (11), whereas the aus subpopulation had the largest average PBL (11 cm). Historically, many of the highest-yielding varieties have been bred within the indica subpopulation [28] , [29] ; accordingly, indica outperformed both aus and tropical japonica in several components of yield as follows: panicle weight, total grain weight and grain number. Interestingly, indica accessions generally had intermediate-sized panicles, but distinctly had the smallest average NL. Despite varying distributions among phenotypes within the subpopulations, all phenotypic and genetic relationships between panicle traits and yield components were largely the same in the Indica and Japonica varietal groups ( Supplementary Figs 3 and 4 ). The highest yielding accessions in our panel never had extreme panicle phenotypes. Subpopulation structure and flowering effects in GWAS The inbreeding nature of rice has led to deep subpopulation structure and considerable linkage disequilibrium (LD), which confounds association studies by reducing mapping resolution and increasing type I error [15] , [17] , [30] . Within our panel, average LD does not decay below an r 2 =0.2 until ∼ 100 kb in indica , 150 kb in aus and 400 kb in tropical japonica ( Supplementary Fig. 5 ). Further, as noted in previous GWAS in rice and Arabidopsis , reproductive phenotypes are particularly susceptible to confounding due to correlations with flowering time and ecological adaptation [16] , [19] , [30] . To address these issues, we used a mixed model to correct for subpopulation structure [31] , integrating the first three PCs as covariates within the model, and performed GWAS across all accessions and within individual subpopulations. In addition, we repeated all analyses with and without use of HD as a phenotypic covariate within the mixed model (see Methods and equation (2)). Detailed association results for every trait, subpopulation and covariate combination are located within the Supplementary Materials ( Supplementary Figs 6–65 and Supplementary Data 1 and 2 ), as well as at www.ricediversity.org . GWAS identified five loci associated with the HD phenotype across the panel, all of which overlap with previously identified HD QTL [32] , [33] , [34] , [35] , [36] , [37] and were detected at low significance ( P <1 × 10 −6 or larger) ( Fig. 3a ). Only one of the peaks, a region on chromosome 2 in the Indica varietal group, overlapped with associations for the panicle traits minimum NL, PL and maximum exsertion thickness ( Fig. 3b ). When HD was used as a phenotypic covariate, GWAS peaks for panicle traits on chromosome 2 were attenuated or eliminated ( Supplementary Figs 9, 12 and 53 ), suggesting that panicle phenology associated with this locus is largely explained by variation in flowering time. In addition, use of the HD covariate reduced the number of significant SNPs associated with panicle traits throughout the genome ( Table 1 ). The effect was most striking within the tropical japonica subpopulation, although a few tropical japonica accessions within the panel are from subtropical regions and may be less adapted for growth in the irrigated tropics ( Supplementary Table 1 ). Many significant SNPs were eliminated from two peaks within the pericentromeric region of chromosome 8 ( ∼ 45 SNPs in tropical japonica and 75 when mapping with all accessions). In addition, many were from PBN traits ( ∼ 130 SNPs), which generally showed improved quantile–quantile plots with the use of the HD covariate ( Supplementary Figs 34–48 ). 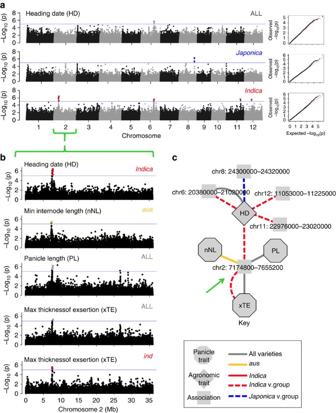Figure 3: Genome-wide association results for HD. (a) Manhattan plots and quantile–quantile plots depicting GWAS results using a mixed model. Associations identified in all accessions, theIndicasubspecies and theJaponicasubspecies are depicted in separate panels. Thexaxis depicts the physical location of SNPs across the 12 chromosomes of rice and theyaxis depicts the −log10(Pvalue). Significant SNPs withP<1 × 10−5are depicted as coloured dots, labelled to match the group in which they were identified (red forIndicaand blue forJaponica). (b) Manhattan plots for chromosome 2. The significant SNP associations for HD in theIndicasubspecies are in LD with significant associations for several panicle traits, depicted in separate panels: minimum NL (nNL) in theaussubpopulation (yellow SNPs); PL and maximum exsertion thickness (TE) across all accessions (grey SNPs); and maximum TE in theindicasubpopulation (ind, red SNPs). (c) An association network summarizing all Manhattan plots inaandb. Traits are labelled with acronyms corresponding tob. LD blocks are labelled with chromosome number and coordinates. Traits and LD blocks containing significant SNPs are treated as nodes and are connected if an LD block contains a significant association for the trait of interest. The colour and style of the edges connecting the trait and associations indicate, which subpopulation or varietal group in which the association was detected. When multiple edges are present between a trait and LD block, a significant association was detected in more than one GWAS. The green arrow indicates the significant peak on chromosome 2 (b), which contains overlapping associations for different types of traits. Figure 3: Genome-wide association results for HD. ( a ) Manhattan plots and quantile–quantile plots depicting GWAS results using a mixed model. Associations identified in all accessions, the Indica subspecies and the Japonica subspecies are depicted in separate panels. The x axis depicts the physical location of SNPs across the 12 chromosomes of rice and the y axis depicts the −log 10 ( P value). Significant SNPs with P <1 × 10 −5 are depicted as coloured dots, labelled to match the group in which they were identified (red for Indica and blue for Japonica ). ( b ) Manhattan plots for chromosome 2. The significant SNP associations for HD in the Indica subspecies are in LD with significant associations for several panicle traits, depicted in separate panels: minimum NL (nNL) in the aus subpopulation (yellow SNPs); PL and maximum exsertion thickness (TE) across all accessions (grey SNPs); and maximum TE in the indica subpopulation ( ind , red SNPs). ( c ) An association network summarizing all Manhattan plots in a and b . Traits are labelled with acronyms corresponding to b . LD blocks are labelled with chromosome number and coordinates. Traits and LD blocks containing significant SNPs are treated as nodes and are connected if an LD block contains a significant association for the trait of interest. The colour and style of the edges connecting the trait and associations indicate, which subpopulation or varietal group in which the association was detected. When multiple edges are present between a trait and LD block, a significant association was detected in more than one GWAS. The green arrow indicates the significant peak on chromosome 2 ( b ), which contains overlapping associations for different types of traits. Full size image Table 1 Genome-wide association results for panicle traits divided by subpopulation and covariate combinations. Full size table These results confirm established pleiotropic relationships between flowering time and inflorescence architecture in rice [38] , [39] , [40] . However, this is not the whole story; including the HD covariate in the mixed model eliminated SNPs associated with several phenotypes, but many SNPs associated with length and width traits were not eliminated and occasionally showed increases in significance ( Table 1 and Supplementary Figs 10d, 30d, 50d, and 51d ). Having properly controlled for the effects of flowering time, we investigated the remaining significant loci associated with panicle phenotypes, which could represent candidates for breeders hoping to tweak panicle architecture to optimize yield performance in the tropics. Thus, unless otherwise noted, all results discussed within the following sections were generated using the HD covariate in the GWAS model. Visualization of complex trait relationships using networks To compare association results across many traits, we constructed ‘association networks’ using the programme Cytoscape [41] . Briefly, significant SNPs were binned into peaks based on physical map position, using a sliding window defined by association significance level and local LD (see Methods and Supplementary Data 3 ). We constructed networks in which traits and peaks were treated as nodes, connected by an edge only when the trait showed significant associations within a given region of the genome. Of the five significant peaks for HD detected in the genome ( Fig. 3a ), only the peak on chromosome 2 overlapped with panicle traits ( Fig. 3b,c ). Association networks provided a visual summary of how peaks were distributed across different traits and allowed us to quantitatively identify regions of the genome associated with multiple phenotypes ( Supplementary Data 4 ). GWAS links panicle trait variation to numerous loci When mapping across all accessions within the panel using the HD covariate, we detected 496 significant SNP associations clustered under 256 peaks located on all 12 chromosomes ( Table 1 ). Many SNPs had small-to-intermediate significance levels ( P <1 × 10 −6 or larger); only 18 SNPs showed a P <1 × 10 −7 and the most significant panicle trait association was for PBL s.d. ( P =8.2 × 10 −9 ; Supplementary Fig. 27 ). These results suggest that panicle morphology is determined by many genes, each with small effect. Although nested phenotypes often shared the same peaks, we detected an increased number of peaks by dividing panicles into sub-traits. For example, we identified 14 significant peaks when mapping for average PBN across all accessions ( Fig. 4 ). Mapping with maximum PBN, minimum PBN and s.d. of PBN (PBNsd) identified an additional 15 peaks on 7 chromosomes that were not detected when mapping with (PBN) ( Fig. 4 and Supplementary Figs 34–39 ). As described above, previous research demonstrated that spikelets located on lower versus upper panicle branches had differential regulation and expression of proteins [27] . Mapping for PBN in the lower and upper halves of the panicle separately ( Fig. 1b ) identified additional five peaks not observed among other primary branch traits ( Fig. 4 ). We also detected an increased number of associations when other traits were subdivided into multiple phenotypes ( Supplementary Figs 17–29, 40–48 and 66 , and Supplementary Data 4 ). These results suggest that partitioning a trait into multiple sub-traits minimizes the variance among raw values, which in turn maximizes the ability to detect differences for that sub-trait. This increases the power of GWAS to detect significant associations. Thus, although clusters of related measurements are highly correlated with one another morphologically and genetically ( Figs 2 and 4 , and Supplementary Figs 3 and 4 ), separating a trait into nested phenotypes appears to resolve the location of small-effect QTL in unique regions of the genome [21] . 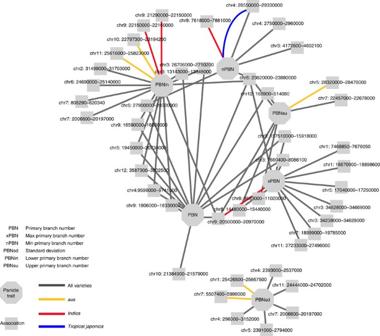Figure 4: Genome-wide association links numerous loci to variation in panicle traits. An association network constructed using PBN traits. Traits and LD blocks containing significant SNPs (P<1 × 10−5) are treated as nodes and are connected if an LD block contains a significant association for the trait of interest. LD blocks are labelled with chromosome number and coordinates. The colour and style of the edges connecting the trait and associations indicate which subpopulation or subspecies in which the association was detected. When multiple edges are present between a trait and LD block, significant associations were detected in multiple populations. Trait abbreviations are as follows: PBN, primary branch number; PBNin, (PBN in lower half of panicle; PBNsu, PBN in upper half of panicle; nPBN, minimum PBN; PBNsd, PBN s.d.; xPBN, maximum PBN. Figure 4: Genome-wide association links numerous loci to variation in panicle traits. An association network constructed using PBN traits. Traits and LD blocks containing significant SNPs ( P <1 × 10 −5 ) are treated as nodes and are connected if an LD block contains a significant association for the trait of interest. LD blocks are labelled with chromosome number and coordinates. The colour and style of the edges connecting the trait and associations indicate which subpopulation or subspecies in which the association was detected. When multiple edges are present between a trait and LD block, significant associations were detected in multiple populations. Trait abbreviations are as follows: PBN, primary branch number; PBNin, (PBN in lower half of panicle; PBNsu, PBN in upper half of panicle; nPBN, minimum PBN; PBNsd, PBN s.d. ; xPBN, maximum PBN. Full size image Subpopulation-specific panicle trait associations Performing GWAS within individual subpopulations identified an additional 107 significant peaks ( Table 1 ). When comparing significant peaks using association networks, we noted that certain types of traits showed enrichment for subpopulation-specific SNPs. For example, although we only identified 10 subpopulation-specific peaks for PBN traits ( Fig. 4 ), we identified 23 peaks for PBL traits ( Supplementary Fig. 66 ). Strikingly, no two subpopulations had a significant peak for the same trait within the same region of the genome ( Supplementary Data 4 ). Only one region of the genome contained peaks for panicle traits identified in two separate subpopulations ( Supplementary Fig. 67 ). Both these observations have been made in rice for other phenotypes, including the traditional breeding phenotype PL ( Fig. 1b ) [15] , [16] , [17] , [19] . The genetic heterogeneity within O. sativa drives trait variation at the subpopulation and subspecies level, and probably explains the phenotypic differences we observe for each subpopulation ( Fig. 2 ). These results also suggest that a sizable portion of the genetic variation responsible for panicle morphology remains isolated within individual subpopulations. Assessing pleiotropy between panicle traits To determine whether relationships between different types of traits (length, width and count) were the result of linkage or pleiotropy, we constructed association networks using every phenotype in the panel. We observed 92 regions of the genome with significant SNPs for more than 1 trait; 10 regions had associations for 8 or more panicle traits ( Supplementary Data 4 ). In most cases, the regions associated with more than one trait were identified when mapping across all accessions in the panel; when mapping within a single subpopulation, the same region was associated with just one or a few traits ( Fig. 5a ). A careful examination of allele frequencies demonstrated that in most cases, the reason for this distribution was the presence of subpopulation-specific alleles that remained significant when all subpopulations were considered together ( Supplementary Data 1 and 2 ). However, we occasionally detected subpopulation-specific associations for multiple traits at one genomic address; an unusual region on chromosome 11 within the aus subpopulation contained associations for nine length and width traits ( Fig. 5a ). 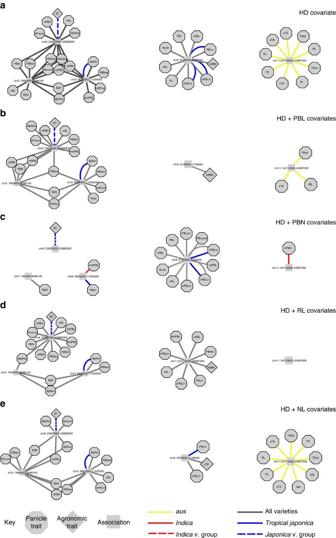Figure 5: Panicle covariates dissect genomic regions containing many associations for different types of traits. Peaks detected using (a) the HD covariate within the GWAS mixed model; (b) HD and PBL covariate; (c) HD and PBN covariate; (d) HD and RL covariate; or (e) HD and NL covariate. Association networks demonstrate that clusters of related traits frequently have overlapping associations within LD blocks. Traits and LD blocks containing significant SNPs (P<1 × 10−5) are treated as nodes and connected if an LD block contains a significant association for the trait of interest. LD blocks are labelled with chromosome number and coordinates. The colour and style of the edges connecting the trait and associations indicate the subpopulation or subspecies in which the association was detected. When multiple edges are present between a trait and LD block, a significant association was detected in more than one GWAS. To simplify networks, acronyms are used. Agronomic traits: booting (BT) and total shoot biomass (totBM). Count traits: PBN, NN and number of branches per internode (BpN). Length traits: PL, RL, PBL and NL. Width traits: thickness of rachis (TR) and thickness of exsertion (TE). In addition to overall trait averages, sub-traits are depicted using acronyms with prefixes and/or suffixes: maximum (x−), minimum (n−), s.d. (−sd), lower (−in) and upper (−su). For example, maximum PBL in the lower half of the panicle (xPBLin). Figure 5: Panicle covariates dissect genomic regions containing many associations for different types of traits. Peaks detected using ( a ) the HD covariate within the GWAS mixed model; ( b ) HD and PBL covariate; ( c ) HD and PBN covariate; ( d ) HD and RL covariate; or ( e ) HD and NL covariate. Association networks demonstrate that clusters of related traits frequently have overlapping associations within LD blocks. Traits and LD blocks containing significant SNPs ( P <1 × 10 −5 ) are treated as nodes and connected if an LD block contains a significant association for the trait of interest. LD blocks are labelled with chromosome number and coordinates. The colour and style of the edges connecting the trait and associations indicate the subpopulation or subspecies in which the association was detected. When multiple edges are present between a trait and LD block, a significant association was detected in more than one GWAS. To simplify networks, acronyms are used. Agronomic traits: booting (BT) and total shoot biomass (totBM). Count traits: PBN, NN and number of branches per internode (BpN). Length traits: PL, RL, PBL and NL. Width traits: thickness of rachis (TR) and thickness of exsertion (TE). In addition to overall trait averages, sub-traits are depicted using acronyms with prefixes and/or suffixes: maximum (x−), minimum (n−), s.d. (−sd), lower (−in) and upper (−su). For example, maximum PBL in the lower half of the panicle (xPBLin). Full size image In general, the same types of traits had overlapping peaks within a given region of the genome. For example, peaks on chromosomes 3 and 8 were associated with PBN and NN traits across all subpopulations, a peak on chromosome 9 was associated with NL and PBL traits, and the peak on chromosomes 11 identified in aus (mentioned above) was associated with overall size traits such as RL, PL and width traits ( Fig. 5a ). This suggested that panicle traits with a shared morphological origin, expansion of tissue versus division of meristems, are more likely to be co-inherited. To test for pleiotropy among panicle traits, we repeated GWAS and sequentially incorporated different panicle traits as a second phenotypic covariate (alongside HD) within the mixed model: PBL, PBN, RL or NL (see Methods, equation (3) and Supplementary Data File 5–10 ). We noted several patterns common to all panicle covariate runs. Although the total number of significant peaks did not drastically change ( Supplementary Table 3 ), peaks identified when mapping across all accessions tended to lose associations with some phenotypes or disappear entirely ( Fig. 5 and Supplementary Figs 68–71 ) and the number of subpopulation-specific peaks increased ( Supplementary Table 3 and Supplementary Figs 68–71 ). In addition, the majority of peaks overlapped with peaks from the HD covariate run ( Supplementary Table 4 ). Interestingly, covariates had different impacts on associations at individual peaks, which mimicked the genetic and phenotypic relationships quantified above ( Fig. 2 and Supplementary Figs 3 and 4 ). The PBL and PBN covariates affected peaks in opposite ways. The PBL covariate eliminated the peak for branch length and NL traits on chromosome 9, yet did not eliminate associations for PBN traits on chromosomes 3, 6 or 8 ( Fig. 5b ). In contrast, the PBN covariate had little effect on the chromosome 9 peak, yet largely eliminated peaks on chromosome 3, 6, 8 and 11 for branch number traits, NN traits and composite traits such as PL or total PBL ( Fig. 5c ). Although the RL covariate eliminated the significant peak in aus on chromosome 11, it did not eliminate the peaks on chromosomes 3, 6, 8 or 9 ( Fig. 5d ); this indicates that genetic variation at certain loci may have an impact on specific stages of panicle development spatiotemporally. Finally, the NL covariate had an impact on peaks similar to the PBL covariate, rather than the RL covariate, indicating that certain peaks may affect NL without affecting RL or overall size of the panicle ( Fig. 5d ). Taken together, these results suggest that specific panicle traits are highly correlated and/or pleiotropic, at least in the environment tested in this study. The way in which panicle covariates ubiquitously had an impact on associations for phenotypes at other loci is also indicative ( Supplementary Figs 68–71 ); small differences in individual traits are likely to be the result of genetic variation that has an impact on a single compensatory network of developmental genes that drives inflorescence morphology as a whole. Relationships among panicle and agronomic trait associations As observed in previous studies, we detected several regions of the genome that contained significant associations for both panicle and agronomic traits. In some cases, agronomic traits were vegetative; for example, a peak on chromosome 1 was associated with PL and flag leaf area, and a peak on chromosome 9 for total shoot biomass overlapped with peaks for many length phenotypes ( Fig. 6 ). Several yield performance traits, such as panicle weight, grain number and 1,000-grain weight (1,000GW) had overlapping peaks with different types of panicle traits as follows: NN, branch length and NL, respectively. Unlike the associations we observed when comparing panicle phenotypes, panicle and agronomic traits never shared exactly the same significant SNPs [19] ( Supplementary Data 1,2 and 5–8 ); rather, significant SNPs were often closely linked within the same LD block (<100 kb). In addition, the use of panicle trait covariates within the mixed model did not eliminate the most significant yield associations ( Supplementary Fig. 72 ). Rather, panicle covariates altered which panicle traits overlapped with agronomic traits. This could suggest that the genetic networks governing agronomic traits operate independently, at least in part, of those responsible for variation in panicle traits detected in the field. 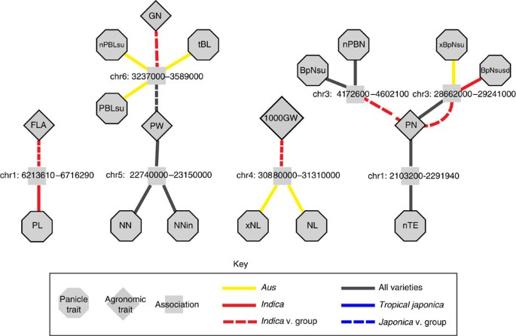Figure 6: Genomic regions containing associations for panicle and agronomic traits when using the HD covariate. Association networks where traits and LD blocks containing significant SNPs (P<1 × 10−5) are treated as nodes and are connected if an LD block contains a significant association for the trait of interest. LD blocks are labelled with chromosome number and coordinates. The colour and style of the edges connecting the trait and associations indicate the subpopulation or varietal group in which the association was detected. When multiple edges are present between a trait and LD block, a significant association was detected in more than one GWAS. To simplify networks, acronyms are used. Agronomic traits: booting (BT) and total shoot biomass (totBM). Count traits: PBN, NN and number of branches per internode (BpN). Length traits: PL, RL, PBL, NL and tip branch length (tBL). Width traits: thickness of rachis (TR) and thickness of exsertion (TE). In addition to overall trait averages, sub-traits are depicted using acronyms with prefixes and/or suffixes: maximum (x−), minimum (n−), s.d. (−sd), lower (−in) and upper (−su). For example, maximum PBL in the lower half of the panicle (xPBLin). Agronomic traits: flag leaf area (FLA), panicle weight (PW), grain number (GN), 1,000GW and panicle number (PN). Figure 6: Genomic regions containing associations for panicle and agronomic traits when using the HD covariate. Association networks where traits and LD blocks containing significant SNPs ( P <1 × 10 −5 ) are treated as nodes and are connected if an LD block contains a significant association for the trait of interest. LD blocks are labelled with chromosome number and coordinates. The colour and style of the edges connecting the trait and associations indicate the subpopulation or varietal group in which the association was detected. When multiple edges are present between a trait and LD block, a significant association was detected in more than one GWAS. To simplify networks, acronyms are used. Agronomic traits: booting (BT) and total shoot biomass (totBM). Count traits: PBN, NN and number of branches per internode (BpN). Length traits: PL, RL, PBL, NL and tip branch length (tBL). Width traits: thickness of rachis (TR) and thickness of exsertion (TE). In addition to overall trait averages, sub-traits are depicted using acronyms with prefixes and/or suffixes: maximum (x−), minimum (n−), s.d. (−sd), lower (−in) and upper (−su). For example, maximum PBL in the lower half of the panicle (xPBLin). Agronomic traits: flag leaf area (FLA), panicle weight (PW), grain number (GN), 1,000GW and panicle number (PN). Full size image Biparental mapping and candidate gene analysis To further assess the genetic architecture of panicle traits, QTL mapping was performed using 168 recombinant inbred lines (RILs) grown in a second environment (see Methods section). By subdividing traits and mapping with nested panicle phenotypes [21] , we were able to dissect several large QTL into overlapping small-effect QTL with varying sizes, significance levels and peak positions; these results mirrored the increased number of GWAS associations detected when mapping with sub-traits ( Fig. 4 ). In total, we identified 129 QTL for panicle phenotypes, 7 for HD and 2 for panicle number ( Supplementary Table 5 ). Strikingly, we observed QTL that overlapped with significant GWAS peaks on 11 out of 12 chromosomes ( Supplementary Figs 83–93 ). Although biparental QTL generally encompassed more than one significant GWAS peak (due to lower resolution of QTL mapping versus GWAS), in several cases the QTL mapping resolution gained by using sub-traits in the RIL population allowed us to narrow in on a single GWAS peak ( Fig. 7 and Supplementary Figs 83, 85–87,90 and 91 ). 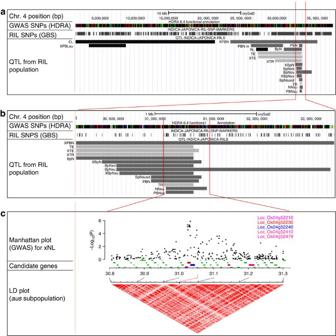Figure 7: Mega-locus on chromosome 4 associated with panicle and yield traits. (a) Physical map of rice chromosome 4 showing the position of SNPs segregating in the GWAS panel (HDRA SNPs) and in the RIL population (genotyping by sequencing (GBS) SNPs). Grey bars indicate the position of QTL identified in the RIL population. Trait acronyms are as follows: 1000GW, PBN, NN, RL, PBL, NL, rachis thickness (TR), exsertion thickness (TE), exsertion length (EL), and number of branches per internode (BpN); sub-traits are depicted using acronyms with prefixes and/or suffixes: maximum (x−), minimum (n−), s.d. (−sd), lower (−in) and upper (−su). For example, PBN in the upper half of the panicle: PBNsu. (b) Zoom-in of 2.5 Mb region of chromosome 4 showing QTLs for panicle traits. (c) Zoom-in of 0.5 Mb region of chromosome 4 showing Manhattan plot, indicating position of GWAS-QTL associated with maximum NL (xNL) and 1000GW. An LD heatmap (D') is depicted in red. Five candidate genes are highlighted as coloured bars below the Manhattan plot:OsKS3=LOC_Os04g52210,OsKS1=LOC_Os04g52230,OsKS2=LOC_Os04g52240,OsMADS31=LOC_Os04g52410 andNAL1=LOC_Os04g52479. Figure 7: Mega-locus on chromosome 4 associated with panicle and yield traits. ( a ) Physical map of rice chromosome 4 showing the position of SNPs segregating in the GWAS panel (HDRA SNPs) and in the RIL population (genotyping by sequencing (GBS) SNPs). Grey bars indicate the position of QTL identified in the RIL population. Trait acronyms are as follows: 1000GW, PBN, NN, RL, PBL, NL, rachis thickness (TR), exsertion thickness (TE), exsertion length (EL), and number of branches per internode (BpN); sub-traits are depicted using acronyms with prefixes and/or suffixes: maximum (x−), minimum (n−), s.d. (−sd), lower (−in) and upper (−su). For example, PBN in the upper half of the panicle: PBNsu. ( b ) Zoom-in of 2.5 Mb region of chromosome 4 showing QTLs for panicle traits. ( c ) Zoom-in of 0.5 Mb region of chromosome 4 showing Manhattan plot, indicating position of GWAS-QTL associated with maximum NL (xNL) and 1000GW. An LD heatmap (D') is depicted in red. Five candidate genes are highlighted as coloured bars below the Manhattan plot: OsKS3= LOC_Os04g52210, OsKS1= LOC_Os04g52230, OsKS2= LOC_Os04g52240, OsMADS31= LOC_Os04g52410 and NAL1= LOC_Os04g52479. Full size image Many genes involved in rice development have been cloned and characterized [6] , [10] . To leverage this resource, we assembled a list of 319 a priori candidate genes ( Supplementary Table 6 ), roughly half of which have been described molecularly, to determine whether any known genes mapped within the expected LD surrounding our GWAS peaks. Based on the most stringent co-localization criteria, we identified ten candidate genes located within 30 kb or less of significant GWAS SNPs (interval of 1–3 genes) ( Table 2 ). Seven of the candidate genes were associated with hormone signalling cascades [42] , [43] , [44] , [45] , [46] , [47] , [48] , [49] , [50] . Using the database RiceFREND [26] , we confirmed that eight of the ten candidates shared a gene co-expression network with at least one other candidate from our a priori gene list ( Supplementary Note , Supplementary Figs 73–82 and Supplementary Data 11 ). In addition, five of the ten a priori candidate genes identified by GWAS were located within QTL identified by the biparental RIL population ( Table 2 and Supplementary Figs 83, 84, 86, 87 and 92 ). Table 2 Candidate genes identified near significant GWAS peaks. Full size table Interestingly, the traits associated with RIL–QTL were sometimes different than the traits associated with GWAS–QTL in the same region. For example, we identified several RIL–QTL for an agronomic trait that overlapped with a GWAS–QTL for a panicle trait, or vice versa ( Supplementary Figs 83–85,87 and 91–93 ). To characterize the relationship between panicle traits and yield components, we examined a region on chromosome 4 that was simultaneously associated with a suite of biparental QTLs for nested panicle phenotypes, a GWAS peak for maximum NL detected in the aus subpopulation and a GWAS peak for 1,000GW detected in the Indica varietal group ( indica + aus subpopulations) ( Fig. 7 ). Within a 300-kb region containing overlap between 14 biparental QTLs and two GWAS peaks, we observed five a priori candidate genes: a cluster of three tandemly linked rice ent-kaurene synthase genes ( OsKS1 , OsKS3 and OsKS3 ) [45] , a rice MADS Box gene ( OsMADS31 ) [44] and NARROW LEAF1 ( NAL1 ) [28] , [51] , [52] , [53] , [54] ( Fig. 7c and Supplementary Data 2 ). Zooming into the region, it became clear that the OsKS gene family fell directly underneath the most significant GWAS SNPs for both maximum NL and 1,000GW ( Supplementary Fig. 94 ), well within the region of intersection between the RIL-QTLs and the GWAS-QTLs. The RiceFREND database [26] also demonstrated that OsKS1 is co-expressed with sucrose synthase ( Supplementary Fig. 76 ). However, although OsMADS31 and NAL1 were further removed from the most significant GWAS–SNPs, neither GWAS nor biparental QTL mapping provided enough resolution to clearly identify which gene(s) are responsible for the phenotypes we observe, nor to distinguish whether multiple genes were acting combinatorially to generate a ‘synthetic’ QTL of larger effect [55] . Linkage between multiple candidate genes within a 300-kb region associated with diverse panicle traits and the yield component 1,000GW warrants further investigation to unravel the potential breeding significance of this region of the rice genome. Although panicles are the grain-bearing organs in rice, breeders have an incomplete picture of the genetic architecture underlying panicle development in different subpopulations and of the relationships between panicle traits and yield performance. Previous GWAS and QTL studies have collected only a limited number of panicle phenotypes and/or assessed plants grown in controlled environments [18] , [19] , [21] . In addition, owing to subpopulation structure and extensive LD in O. sativa , many studies have evaluated large panels of diverse germplasm to increase GWAS mapping resolution [16] , [17] , [19] , [23] . Although these approaches improve resolution, they considerably confound panicle trait associations with loci responsible for flowering and ecological adaptation [30] , [56] , [57] . We demonstrate that with proper controls for subpopulation structure and flowering, it is possible to detect GWAS peaks associated with reproductive phenotypes and identify SNPs closely associated with a priori candidate genes from pathways known to regulate rice plant architecture ( Table 2 ). The success of our GWAS was undoubtedly due to a combination of phenotypic resolution and use of a high-quality SNP data set from the HDRA [20] . Thus, for breeders and biologists interested in quantifying the genetic architecture of traits, medium-size populations can be used to detect both large- and small-effect loci in the field, provided dense marker data are complemented with precise phenotyping methodologies. We document quantitative variation among panicle traits within and across rice subpopulations and suggest that, in contrast to maize, no one aspect of panicle size or morphology has been severely aggrandized or optimized during domestication. Instead, panicle architecture appears to comprise multiple correlated components of relatively small effect that interact and compensate for one another during development. The number of panicle associations we detect is consistent with the number of genes reported to be expressed during rice [58] , [59] and maize inflorescence development [60] , and we hypothesize that combinations of alleles not detected by GWAS in this study may further enhance subpopulation-specific morphology. Thus, although the underlying genetics governing rice panicle traits are highly subpopulation-specific, overall phenotypic outcomes appear surprisingly similar—even to wild relatives [9] . Gene expression levels have been shown to directly affect flowering time in rice [61] . Our ability to detect distinct associations when mapping for nested traits such as those from lower versus upper panicle traits suggests that we may be capturing genes with spatiotemporal expression differences. Peaks independently associated with length or count traits, or that were preferentially eliminated by certain panicle covariates, are particularly promising for breeders; they may tag genetic variation that can be targeted for selection to tweak individual traits without affecting other aspects of panicle architecture. In keeping with this perspective, we note that the highest yielding indica accessions in our panel have characteristically intermediate panicle phenotypes and the smallest NL (Fig. 2), a trait linked to rice yield performance [12] . However, deep genome-wide differentiation between subpopulations means that a gene can have different phenotypic consequences in different genetic backgrounds [18] , [19] . Thus, it may only be possible to predict the impact of genetic variation associated with panicle traits when operating within a subpopulation, although recombination across subpopulations provides opportunity to drive transgressive phenotypes with extraordinary outcomes. Within the public breeding community, there have been two major initiatives over the past 70 years to boost yield by optimizing independent phases of rice development. The first occurred during the Green Revolution, when breeders successfully leveraged a large-effect allele of SEMIDWARF1 ( SD1 ) and optimized vegetative architecture without drastically changing panicle phenotypes [42] ; our detection of discrete associations for agronomic traits unaffected by panicle trait covariates reconfirm that critical rice genes may operate only during specific stages of development [6] . The second breeding initiative, development of the ‘New Plant Type’ ideotype, attempted to boost yield by simultaneously selecting for increased panicle size (sink) and photosynthetic capacity (source) [62] . This was done using introgression of genomic regions associated with large panicles and low-tillering from tropical japonica into indica varieties [63] , [64] . Given the quantitative nature of panicle development that we detected within and between indica and tropical japonica , it is not surprising that the New Plant Type initiative successfully generated large panicle phenotypes but failed to achieve desired combinations of sink and source traits that generate high-yielding varieties [63] , [64] . The sheer number and non-additive behaviour of loci contributing to panicle morphology suggest that physiologically optimizing panicle architecture for grain filling and yield per se will probably involve managing a highly interactive network or trait complex. This will require integrating quantitative tools and strategies, such as those used in this study, into model-based crop improvement pipelines incorporating genomic selection. That being said, targeted introgression of key genomic regions encompassing specific combinations of beneficial alleles in the form of a complex or ‘synthetic’ QTL holds great promise as a strategy for coordinately improving the suites of traits that are essential for resilience and yield improvement [55] . The NAL1-OsKS1 megalocus on chromosome 4 is of particular interest for rice breeding because it is rich in allelic variation and multiple studies have demonstrated yield improvement using introgression of Japonica alleles into Indica varieties [28] , [51] , [52] , [54] . These findings raise interesting questions about the value of subpopulation-specific allele introgression, genotype by genotype interaction and the role of linked genes that hitchhike along with a target introgression [55] . NAL1 is hypothesized to have been a target of selection during rice domestication [54] and is known to encode a plant-specific protein involved in control of the cell cycle, cell division and polar auxin transport, with pleiotropic effects on vascular patterning, flag leaf area, leaf chlorophyll content, photosynthetic efficiency, panicle size, panicle branching, spikelet number and overall plant architecture [28] , [51] , [52] , [53] , [54] . Less is known about the potential contribution of OsKS1 , which is tandemly linked with two of its homologues ( OsKS2 and OsKS3 ) in the region and catalyses an early step in gibberellin biosynthesis, with mutant alleles leading to dwarfing phenotypes in both vegetative and reproductive tissue [45] , or OsMADS31 , which is ubiquitously expressed throughout panicle development and the first stages of seed formation [44] . The opportunity to optimize linked arrays of alleles that are co-inherited in applied rice breeding represents an exciting new research horizon. The phenotyping methods and mapping resolution presented in this study provide us with the ability to hypothesize the existence of numerous complex QTL that merit further dissection using expression QTL mapping [65] or molecular studies using targeted genome editing. By identifying, understanding and integrating subpopulation-specific variation using a combination of approaches, breeders may one day close the gap between panicle development and yield optimization in rice. GWAS germplasm selection A collection of 1,568 accessions representing the five major subpopulations in O. sativa was recently genotyped for 700,000 SNPs using an HDRA [20] . We wished to maximize the diversity among rice accessions with HDRA genotypes and minimize confounding effects relating to poor adaptation for growth in the tropics. Most accessions were selected from three rice subpopulations (63 aus , 84 indica , 79 tropical japonica , 11 admixed Japonica , 3 temperate japonica and 2 admixed accessions). Detailed information regarding accessions is located within Supplementary Table 1 . RIL population The RIL population used in this study was originally developed from a wide cross between IR64 ( Indica ) and Azucena ( Japonica ), followed by single-seed descent in the greenhouse at Institut de Recherche pour le Développement in Montpellier, France. Both IR64 and Azucena were included the diversity panel used for GWAS ( Supplementary Table 1 ). As described previously, the RILs were genotyped using genotyping by sequencing for 30,984 SNPs at Cornell University [66] . Population structure The PC analysis was conducted using the svd() function in R [67] (version 3.1.0), calculated using SNPs present in all accessions. The Bayesian clustering programme fastStructure was used to calculate varying levels of K ( K =1–10) and the command chooseK.py was used to identify the model complexity that maximized the marginal likelihood ( K =8). Supplementary Fig. 1a was generated using the programme distruct [68] . Genome-wide LD was estimated using pairwise r 2 between SNPs, which was calculated using the --r2 --ld-window 99999 --ld-window-r2 0 command in PLINK [69] (version 1.07). Phenotyping details For the GWAS diversity panel, three replications of each variety were evaluated during the 2013 dry season (January–May) at the International Rice Research Institute in Los Baños, Philippines in a randomized block design under flooded paddy conditions. Each replication consisted of a two-row plot 4.6 m in length, with 0.2 m between plants and 0.3 m between rows. Panicle traits, HD and booting date were collected on all 242 accessions within the panel. All other yield components were collected on 136 randomly sampled accessions from the indica , aus and tropical japonica subpopulations ( Supplementary Table 1 ). Detailed descriptions of all phenotypes, acronyms and measurement methods are presented in Supplementary Table 2 . Raw phenotypes and trait averages used for genetic mapping are stored in Supplementary Data 12 and 13 . Three plant replicates for each of the 168 RILs used for QTL mapping were grown in the Guterman greenhouse in Ithaca, New York, during summer 2012 using a pseudo-randomized block design that accounted for extreme plant height differences [21] ; the population is an expansion in both the number of lines and number of phenotypes over that described in Crowell et al. [21] HD was measured as the point at which the first panicle on a plant had emerged 50% from the flag leaf sheath. Panicle number was measured as the total number of panicles on a plant. When available, 5 panicles per plant were photographed ( n =15 panicles per RIL) using the PANorama imaging protocol described below [21] . Raw phenotypes and trait averages used for genetic mapping are stored in Supplementary Data 14 and 15 . Panicle imaging protocol Following the PANorama imaging protocol [21] , 3,443 images were collected and analysed using a pixel to length conversion of 114.5 pixels per cm. PANorama1.0 contained phenotyping capabilities for 18 major traits, which were calculated via image segmentation and subdivision of panicle axes [18] . Additional, nested phenotypes used in this study (that is, subdivision of the panicle axes into upper and lower halves) were calculated from measurements extracted after the image segmentation and skeletonization process, and thus did not require alternation to the algorithms implemented in PANorama1.0. Detailed descriptions of these phenotypes are available in Supplementary Table 2 . An updated version of PANorama containing all nested phenotypes used within this study, PANorama2.0, is available for download at sourceforge.net/panorama1 . Phenotype statistical analyses Histograms, boxplots, correlations and GWAS analyses were constructed using phenotypic grand means for each variety. P- values for Pearson’s correlation coefficients were calculated with a two-sided t -test using the cor.test() function in R [67] . We provide pseudo-heritability of several phenotypes, described here as ‘AD heritability’, using the Methods described in Spindel et al. [25] The restricted maximum likelihood estimate of the genetic variance was calculated using the mixed.solve() function in the R package rrBLUP (version 4.3) and the value was divided by the total phenotypic variance. Broad sense heritability (H) for each phenotype was estimated using repeatability among phenotypic measurements, calculated as the variance among variety grand means divided by the total phenotypic variance of raw trait values. The best linear unbiased predictors (BLUPs) for genetic values were calculated using the mixed.solve() function in the R package rrBLUP (version 4.3). P- values for genetic correlation coefficients between BLUPs were calculated with a two-sided t -test using the cor.test() function in R [67] . GWAS mapping EMMAX was used to calculate the linear mixed model and significance levels within the GWAS model [31] . For all GWAS runs, within subpopulations or across all accessions, we used the equation: For GWAS runs incorporating HD as a covariate: For GWAS runs incorporating a panicle trait as a covariate: where Y and X represent the phenotype and SNP genotype vectors, respectively; P is a matrix containing the residuals of the first three PCs; HD represents a vector of the HD phenotype; and PAN represents a vector of the panicle phenotype used within the run (RL, PBN, PBL or NL depending on the run). For genotypic and environmental random effects, respectively, μ ∼ N (0, σ 2 g K ) and ɛ ∼ N (0, σ 2 e I ), where K is an identity by state kinship matrix accounting for pairwise relatedness between accessions. SNP marker filtering (minor allele frequency=0.1 and genetic missingness=0.3) and identity by state matrix calculations were performed using PLINK [69] . As yield components were collected on a subset of the accessions within our panel ( Supplementary Table 1 ), we performed GWAS for these traits within the Indica and Japonica subspecies rather than in the individual subpopulations, to maximize our power to detect loci. We noted that certain traits were more susceptible to confounding than others, especially when performing GWAS across subpopulations using the entire panel of accessions. To correct for these issues, we systematically diagnosed the quantile–quantile plots for every trait–subpopulation–covariate combination and used logarithmic transformations on non-normal phenotypes ( Supplementary Table 2 ). The significance threshold was set at P <1 × 10 −5 for every trait and was similar to the false discovery rate [20] . QTL mapping Using R/QTL (version 1.24.9), QTL mapping was performed as described in Crowell et al. [21] . Briefly, QTL were identified using Haley–Knott regression and the significance threshold was set using 1,000 permutations. We then scanned for QTL, condition on peaks that had already been detected. Finally, forward selection and backward elimination were used to refine QTL locations. All phenotypic distributions were systematically diagnosed for normality using a Shapiro–Wilkes test and non-normal phenotypes were transformed logarithmically before mapping. For highly non-normal phenotypes that could not be corrected using transformation, a non-parametric QTL model was used. Supplementary Table 5 contains a list of QTL results, including information regarding transformations and QTL model used on a per trait basis. We also provide visual summaries of significant QTL intervals using the track feature in the UCSC Genome Browser ( Supplementary Figs 83–93 ) ( www.genome.ucsc.edu ). Association networks Significant SNPs were binned together into peaks using a sliding window based on the decay of a LD using the PLINK [67] command --clump-p1 0.00001 --clump-p2 0.0001 --clump-r2 0.3 --clump-kb 150 --clump-allow-overlap. Thus, for every SNP with P <1 × 10 −5 , pairwise r 2 -values were calculated between surrounding SNPs that (1) fell within 150 kb and (2) had a P <1 × 10 −3 ; any two SNPs meeting this criteria that also shared an r 2 ≥0.3 were clumped into bins. All significant SNPs within the study were used in the construction of bins, regardless of the traits with which they shared associations. In addition, any bins sharing overlapping borders after using the PLINK clump command were collapsed into a single bin. Singleton, significant SNPs (<1 × 10 −5 ) were discarded if no other SNP within the LD window was<2.5 × 10 −4 . To construct association networks, traits and their corresponding bins were treated as nodes within the programme Cytoscape [41] (version 3.1) and edges were labelled by the subpopulation in which the trait association was identified. Candidate gene analyses A list of 319 candidate genes was assembled using a literature review and BLAST searches for candidate gene homologues ( Supplementary Table 6 ). Single gene coexpression networks for the a priori candidate genes in Table 2 were constructed in RiceFREND [26] ( http://ricefrend.dna.affrc.go.jp/ ) using the settings displayed alongside the HyperTree in Supplementary Figs 73–82 . Raw RiceFREND data are available in Supplementary Data 9 . LD plots and r 2 -values for candidate gene zoom-ins were constructed using Haploview [70] (version 4.2). How to cite this article: Crowell, S. et al. Genome-wide association and high-resolution phenotyping link Oryza sativa panicle traits to numerous trait-specific QTL clusters. Nat. Commun. 7:10527 doi: 10.1038/ncomms10527 (2016).